The tobacco genome sequence and its comparison with those of tomato and potato The allotetraploid plant Nicotiana tabacum (common tobacco) is a major crop species and a model organism, for which only very fragmented genomic sequences are currently available. Here we report high-quality draft genomes for three main tobacco varieties. These genomes show both the low divergence of tobacco from its ancestors and microsynteny with other Solanaceae species. We identify over 90,000 gene models and determine the ancestral origin of tobacco mosaic virus and potyvirus disease resistance in tobacco. We anticipate that the draft genomes will strengthen the use of N. tabacum as a versatile model organism for functional genomics and biotechnology applications. Common tobacco ( Nicotiana tabacum ) is one of the most widely cultivated non-food crops worldwide and is grown in ~120 countries [1] . It belongs to the Nicotiana genus, which is named after Jean Nicot de Villemain who, in 1560, became the first person to import these plants from the Americas to Europe. The term Nicotiana was originally used by Adam Lonitzer to describe tobacco plants in 1630 (ref. 2 ) and in 1788 by Carl von Linné (Linnaeus) to designate the entire genus [3] . Over 75 naturally occurring Nicotiana species, including 49 native to America and 25 native to Australia [4] , have been classified by Goodspeed [5] and Knapp [6] . Most commercial tobaccos cultivated today belong to the species Nicotiana tabacum L., for which >1,600 N. tabacum cultivated varieties (cultivars) are listed in the National Plant Germplasm System [7] . The three most commonly used tobacco types are Flue-Cured (or Virginia), Burley and Oriental, which are traditionally grown and harvested under different agricultural practices [8] . Tobacco is a model plant organism for studying fundamental biological processes [9] , and is the source of the BY-2 plant cell line, which is a key tool for plant molecular research [10] . It is also used as a model for plant disease susceptibility, which it shares with other Solanaceae plants including potato, tomato and pepper. Diseases affecting tobacco include the tobacco mosaic virus (TMV), the tobacco vein mottling virus (TVMV), the tobacco etch virus (TEV), and the potato virus Y (PVY); the TN90 variety of tobacco, which we sequenced here, is notable in that is has been bred to resist these viral infections. Considerable interest has centred on understanding the origin, organization and evolution of the N. tabacum genome. Tobacco stands out as a complex allotetraploid with a large 4.5 Gb genome with significant proportion (>70%) of repeats [11] , [12] . As a species, N. tabacum (2 n =4 x =48) evolved through the interspecific hybridization of the ancestors of Nicotiana sylvestris (2 n =24, maternal donor) and Nicotiana tomentosiformis (2 n =24, paternal donor) about 200,000 years ago [13] . Because of its complexity and importance, the tobacco genome is a target for the SOL-100 sequencing project [14] , which aims to decipher the genomes of the most important Solanaceae species. The genome sequences of modern varieties of ancestral species were recently reported [15] , and limited evidence suggests that Nicotiana otophora is an alternative paternal donor [16] , [17] . In this report, however, we demonstrate that this is unlikely because of the higher sequence identity of the N. tabacum T-genome with that of N. tomentosiformis . We show the chromosomal rearrangements between the ancestral and tobacco chromosomes, and provide an explanation for an apparent genome reduction following the hybridization. In addition, we present a genomic comparison of tobacco to two other solanaceous species, tomato and potato. Significant chromosomal reshuffling is clearly observed for all chromosomes despite the conservation of their overall count, confirming previous reports [18] . Tobacco’s rich metabolism (involving >4,000 chemical components) and exceptional ability to express proteins (>40% of its dry weight) have prompted numerous initiatives to harness its potential for the production of biologically active substances [19] . Here, we describe the major alkaloid biosynthesis pathway in Nicotiana species, as well as glutamate/aspartate pathways in the three main tobacco types. In this work, we sequence the genomes of key representatives of the three major types of tobacco and combine them with genetic and physical maps of tobacco [20] , [21] . We verify genome assembly accuracy by mapping transcriptomics and Exon Array [22] data of corresponding varieties, we assess the consistency of assemblies and published physical and genetic maps, and we compare N. tabacum S- and T-genomes with those of N. sylvestris and N. tomentosiformis . Sequencing and assembly Genome assembly of polyploid species, such as coffee ( Coffea arabica ), potato ( Solanum tuberosum ) and wheat ( Triticum aestivum ) is challenging. Even the assembly of the relatively small Brassica napus genome (1.2 Gb), which has well-annotated ancestral reference sequences, is still ongoing [23] . We sequenced the genomes of three inbred varieties of the allotetraploid N. tabacum , K326 (Flue-cured), TN90 (Burley) and Basma Xanthi (BX, Oriental), using a whole-genome shotgun sequencing approach with 100 bp Illumina HiSeq-2000 paired-end and mate-pair reads. The size of the tobacco genome has been estimated to be 4.46 Gb by flow cytometry using the fluorochrome propidium iodide [24] and 5.06 Gb by Feulgen microdensitometry [13] . Our estimations based on 17-mer depth distributions of raw sequencing reads [25] , [26] were 4.41 Gb for N. tabacum TN90, 4.60 Gb for N. tabacum K326 and 4.57 Gb for N. tabacum BX. These represent a reduction of 4–8% of the tobacco genome compared with the sum of the ancestral N. sylvestris (2.59 Gb) and N. tomentosiformis (2.22 Gb), which is consistent with the previously published downsizing of 3.7% (ref. 13 ). The genomes were assembled using SOAPdenovo 1.05 (ref. 27 ) with a k-mer of 63 by creating contigs from the variety-specific paired-end reads, scaffolding them with Nicotiana mate-pair libraries, closing the scaffolding gaps using variety-specific paired-end reads and filtering gap closing artifacts. 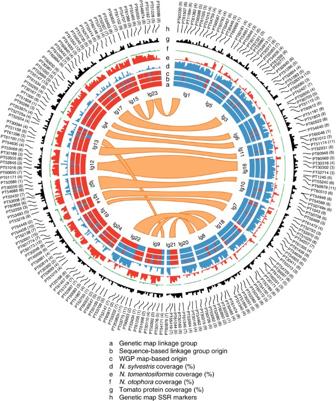Figure 1: Tobacco genome. Blue and red represent features of S and T origins in theNicotiana tabacumTN90 genome, respectively. Track a indicates the origin of the linkage group previously determined by SSR amplification. Track b shows the assignment of the linkage group origin based on sequence identity withN. sylvestris,N. tomentosiformisandN. otophora. Track c shows the origin of the WGP physical map contig used for super-scaffolding. The blue, red and green histograms (tracks d, e and f, respectively) indicate the percentage of each 2 Mb region covered by anN. sylvestris,N. tomentosiformisorN. otophorasequence of at least 1,000 bp and 98% identity. Track g shows the density of coding regions identified by mapping of reference tomato proteins. Track h gives the position of SSR markers mapped to the genome sequences. The centre links regions of theN. tabacumgenome based on sequence homology, as determined by reference tomato proteins mapping at two locations. The resulting final assemblies, described in Table 1 , each amount to 3.7 Gb, representing a coverage of >80% of the tobacco genome. The remaining ~20% is likely to consist of repetitive regions that could not be resolved using the short read de novo shotgun approach. This represents a great improvement from the previous publicly available tobacco genome assembly ( ftp://ftp.solgenomics.net/tobacco_genome/assembly/ ), which contains 294,750 sequences (8.5% of the tobacco genome). We also sequenced libraries from N. otophora to investigate its contribution to N. tabacum . Table 1 Assembly statistics of tobacco genomes. Full size table We evaluated the quality of the scaffolding by mapping the assembly scaffolds to long BAC sequences (altogether 1.8 Mb) obtained from Nicotiana tabacum Hicks Broadleaf. We did not observe any sequence inversions due to scaffolding, and identified only three cases where a contig was not incorporated in a scaffold and remained as singleton ( Supplementary Data 1 ). We also identified 13 cases of insertions or deletions. Altogether this represents 8.6 structural differences per megabase, if we assume that the Hicks Broadleaf sequence is the same as the TN90, K326 and BX sequence for the selected BACs. The sequence-based Whole Genome Profiling (WGP) physical map was used to super-scaffold each genome assembly, and simple sequence repeats (SSRs) were mapped to super-scaffolded assemblies to anchor them to the 24 tobacco linkage groups. This resulted in 84% of the de novo assembly of TN90 being anchored to the WGP physical map (83 and 84% for K326 and BX, respectively), and 19% to the genetic map (17 and 16% for K326 and BX, respectively). Figure 1 shows the composition of the N. tabacum TN90 genome anchored to the linkage groups of the tobacco genetic map. Figure 1: Tobacco genome. Blue and red represent features of S and T origins in the Nicotiana tabacum TN90 genome, respectively. Track a indicates the origin of the linkage group previously determined by SSR amplification. Track b shows the assignment of the linkage group origin based on sequence identity with N. sylvestris , N. tomentosiformis and N. otophora . Track c shows the origin of the WGP physical map contig used for super-scaffolding. The blue, red and green histograms (tracks d, e and f, respectively) indicate the percentage of each 2 Mb region covered by an N. sylvestris , N. tomentosiformis or N. otophora sequence of at least 1,000 bp and 98% identity. Track g shows the density of coding regions identified by mapping of reference tomato proteins. Track h gives the position of SSR markers mapped to the genome sequences. The centre links regions of the N. tabacum genome based on sequence homology, as determined by reference tomato proteins mapping at two locations. Full size image The three methods for assigning an ancestral origin to the linkage groups, SSR amplification in N. sylvestris and N. tomentosiformis [20] , sequence identity with donor species and using the WGP physical map [21] , are concordant. The latter two confirmed the previously reported colour inversion in linkage group 22 (ref. 21 ), and the central part of Fig. 1 clearly shows the correspondence between regions of different ancestral origins within regions of the N. tabacum genome linked by sequence homology. By mapping SSR markers to the sequenced genomes of N. tabacum K326, TN90 and BX, we were able to predict SSR length differences between the three varieties. When comparing TN90 to K326, 57% of the predictions obtained exactly matched experimental measurements, and 10% had only 2-bp differences. The larger differences observed between experimental and in silico SSR measurements are likely to be caused by difficulties in resolving the SSR using short read assembly. We used sequence identity to assign an ancestral origin to each 2-Mb region. The only region for which N. otophora appears as the most likely ancestor is at the end of linkage group 14 ( Supplementary Fig. 1 ), indicating that if it contributed to the N. tabacum genome, then only marginally. This observation favours the hypothesis that the predominant paternal donor was N. tomentosiformis [28] . We evaluated the completeness of our assemblies by mapping reference gene sequences to each genome using BLAT [29] ( Supplementary Table 1 ). For this we used NCBI and SGN tobacco Unigene constructs, as well as the SGN tobacco transcriptome [30] . We also used the coding sequences of tomato (ITAG v2.3) and potato (PGSC v3.4). We mapped 82–86% of the tobacco transcriptome; the remainder is likely to consist of genes spanning different genome sequences that have not yet been scaffolded. Between 50–59% of the Unigene constructs from NCBI and SGN could be mapped, presumably reflecting sequence diversity in the Unigene set [31] . Approximately 60% of the tomato and potato coding sequences could be mapped to the genomes, which compares favourably with the rate of transcript mapping to the Nicotiana benthamiana genome [31] (56.5 and 58.5% for tomato and potato, respectively). In 92.8% of the cases, the best possible alignment of a tomato protein overlaps with a tobacco gene model from our TN90 transcriptome (nine tissues). The genetic and physical map anchoring results as well as alignment to the N. sylvestris and N. tomentosiformis genomes confirmed the quality of the three N. tabacum genome assemblies. Synteny with other Solanaceae The linkage groups from the genetic maps of both N. tomentosiformis and N. acuminata [18] , and the results of SSR amplification in N. tomentosiformis and N. sylvestris [20] , were used to show rearrangements that are found in tobacco ( Supplementary Data 2 and 3 ). 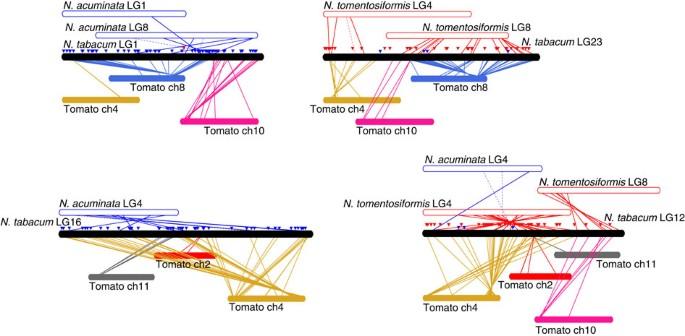Figure 2: Synteny betweenNicotiana tabacum,Nicotiana tomentosiformisandNicotiana acuminatagenetic linkage groups and tomato chromosomes. Links between tomato and tobacco are based on the mapping of tomato proteins to linkage group-anchored tobacco sequences. Note that not all regions identified by this method should necessarily be considered as syntenic. Links between tobacco andN. tomentosiformis(red) andN. acuminata(blue) are based on shared SSR (full lines) and COSII (dotted lines) markers. Triangles indicate the amplification of the corresponding SSR inN. tomentosiformis(red) orN. sylvestris(blue). Figure 2 illustrates one such rearrangement, where part of linkage groups 4 and 8 of N. tomentosiformis are fused to give N. tabacum linkage groups 12 and 23, whereas N. acuminata linkage groups 4 and 8 did not fuse, and gave N. tabacum linkage groups 16 and 1, respectively. Figure 2: Synteny between Nicotiana tabacum , Nicotiana tomentosiformis and Nicotiana acuminata genetic linkage groups and tomato chromosomes. Links between tomato and tobacco are based on the mapping of tomato proteins to linkage group-anchored tobacco sequences. Note that not all regions identified by this method should necessarily be considered as syntenic. Links between tobacco and N. tomentosiformis (red) and N. acuminata (blue) are based on shared SSR (full lines) and COSII (dotted lines) markers. Triangles indicate the amplification of the corresponding SSR in N. tomentosiformis (red) or N. sylvestris (blue). Full size image The synteny between the genomes of N. tabacum TN90, K326 and BX and those of tomato and potato was evaluated at the protein level by mapping tomato and potato proteins to tobacco sequences anchored to the linkage groups of the genetic map [20] to detect homologous genes ( Supplementary Data 2 and 3 ), and by detecting further homologous DNA blocks in genomes masked for repeats ( Supplementary Data 4–7 ). Similar results were obtained using MCScanX [32] , which is a toolkit specifically designed for the detection and analysis of gene synteny and collinearity ( Supplementary Data 8 and 9 ). Not all the regions identified by either of these methods should be considered as truly syntenic, as some of them rely only on a limited number of anchors. Likewise, additional syntenic regions are likely to exist, which cannot be detected by the methods used here. Nevertheless, these approaches confirm results reported earlier based on COSII (ref. 18 ) and SSR markers [20] . Repetitive elements in the genomes The repeat content of the N. tabacum K326, TN90 and BX genomes is summarized in Supplementary Table 2 . Between 72 and 79% of the sequenced genomes are reported as repeat elements by RepeatMasker. This estimation is lower than that reported for barley (84%) and close to the original estimate (~80%) by Zimmerman [11] . Based on the amount of the sequenced genome covered by repeats, we evaluated the DNA portion of the tobacco genome containing non-repeat coding regions to about 1 Gb. This is equivalent to the sum of the same DNA portion from the descendants of both ancestral genomes. The observed 4–8% reduction in genome size is thus likely to have occurred in the repetitive region of the genome. The sum of the genome sizes from the descendants of both ancestors is of 5.04 Gb, N. sylvestris accounting for 53% of it, and N. tomentosiformis for 47%. The tobacco scaffolds to which an origin could be assigned show 55–57% of S origin and 43–45% of T origin. The genome reduction thus is likely to have been more important in the T part of the genome than in the S part, which corresponds to what was reported by Renny-Byfield et al. [12] The reported assemblies of three tobacco varieties cover >80% of the genome, which is comparable to that for smaller diploid genomes (76–90%) [25] , [33] and for the smaller (3 Gb) allotetraploid N. benthamiana (81–87%) [30] , [34] . They represent some of the largest assembled plant genomes together with barley (5.1 Gb) [35] , Norway spruce (20 Gb) [36] and the partial wheat genome (17 Gb) [37] . Contrary to other allotetraploid genomes, for which ancestral information is either not available ( N. benthamiana ) or limited (wheat), the ancestral origin of the tobacco sequences was identified and confirms previously reported assignments based on genetic markers [20] and the physical map [21] . Tobacco root and leaf transcriptome analysis For each variety, three biological replicates were obtained from roots and leaves, which are two metabolically highly active tobacco tissues. In addition, nine tissues were sampled for TN90, so as to get good coverage of the gene regions. 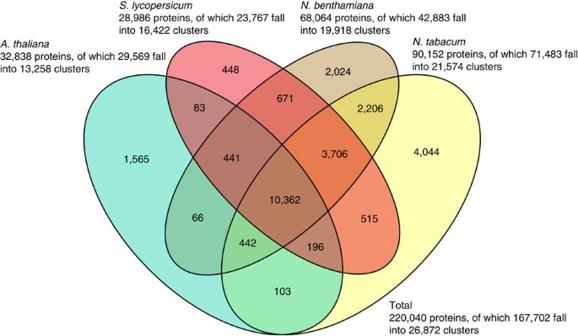Figure 3: Protein clusters shared between tobacco and other increasingly more distant species phylogenetically. Nicotiana benthamianais a representative of the Nicotiana genus,Solanum lycopersicum(tomato) is a representative of the Solanum genus andArabidopsis thalianais a representative of the eudicotyledons. For each RNA-Seq sample, 86.5–94.7% of reads were mapped to the genome of the corresponding variety ( Supplementary Table 3 ). Using RNA-seq data from two tissue types, we generated gene models for each of the three varieties, the gene number estimate being 81,000 for TN90 ( Supplementary Table 4 ). Using data from nine tissue samples increases this estimate by 14.7% to >93,000 genes. Of the 134,694–188,510 transcripts, approximately half this number of unique open reading frames can be found ( Supplementary Table 4 ). These numbers do not represent the whole transcriptome of tobacco, as we sampled RNA from only nine tissues, and hence will be missing transcripts not expressed in any of them. For the root and leaf transcriptomes, gene ontology (GO) terms could be assigned by InterProScan [38] to ~40,000 proteins (from ~28,000 genes) ( Supplementary Table 5 ); for the nine tissue samples, this number increases to >50,000, although there is notable increase in the number of unique GO terms assigned. A recent analysis of 454 N. sylvestris , N. tomentosiformis and N. tabacum next-generation sequencing transcriptomes showed neither differences in gene expression nor the creation of a new function for homoeologous genes between N. tabacum S- and T genomes [30] . Similarly, we found no new genes or new functionality of existing genes in the three varieties. We analysed the GO term enrichment for differentially expressed genes in each tissue. Photosynthesis- and biosynthetic-related genes were highly expressed and enriched in leaf tissue, as were genes involved in oxidation–reduction processes ( Supplementary Fig. 2 ). Root tissue has a very distinctive profile of upregulated genes ( Supplementary Fig. 3 ). Besides lipid transport and regulatory gene overexpression, lignin and cell wall metabolism genes were prominent. Moreover, defence and oxidative stress response genes were heavily upregulated, which may be related to cell death processes apparent from the expression profile. The overexpression of ‘pollination’ genes reflects the electronic annotation of several upregulated proteins within the PFAM domain PF00954, the so-called ‘S locus glycoprotein-like’ domain. While this protein family is best known for being involved in the pollination process, some members are involved in defence response regulation [39] . It is thus more likely that the proteins identified here are involved in defence, rather than in pollination. We used OrthoMCL to analyse the functional overlap between tobacco and three other, increasingly divergent plant species: N. benthamiana as a further representative of the Nicotiana genus, Solanum lycopersicum (tomato) as a further species in the Solanaceae family and Arabidopsis thaliana , another species in the eudicotyledons ( Fig. 3 ). The bulk of the protein clusters are shared between all dicotyledons (10,362), we observed 2,024 and 4,044 clusters specific to N. benthamiana and N. tabacum , respectively, and 2,206 Nicotiana-specific clusters shared between both species. We also observed 3,706 clusters shared between all Solanaceae but not with Arabidopsis. Figure 3: Protein clusters shared between tobacco and other increasingly more distant species phylogenetically. Nicotiana benthamiana is a representative of the Nicotiana genus, Solanum lycopersicum (tomato) is a representative of the Solanum genus and Arabidopsis thaliana is a representative of the eudicotyledons. Full size image Classical tobacco pathways We extracted the sequences of biochemical pathway enzymes and observed copy numbers and expression in roots and leaves under different growth conditions ( Supplementary Note 1 ). No major differences in gene expression were observed, but one new putrescine N-methyltransferase gene was identified in the alkaloid pathway in addition to the four already reported [40] . Furthermore, the two quinolinate phosphoribosyltransferase (QPT) genes of S origin were not found in N. tabacum K326 ( Supplementary Table 6 and Supplementary Table 7 ). Most described alkaloid genes are expressed in roots where most alkaloids are synthesized; however, some transcripts from AO , QPT , QS and MPO genes were also detected in leaf, suggesting that they have different functions ( Supplementary Fig. 4 and Supplementary Note 1 ). In addition, we have mapped the putative steroidal alkaloid biosynthesis genes from Nicotiana genomes to the syntenic regions recently discovered on chromosomes 7 and 12 of S. lycopersicum [41] . In N. tabacum we identified two copies of each region, corresponding to their ancestral origin, indicating that these regions are conserved within Nicotiana species ( Supplementary Fig. 5 ). For Burley tobacco, which is known for its high nitrogen requirement, nitrogen assimilation is stronger than for Flue-cured tobacco ( Supplementary Fig. 6 ). We therefore compared the number and expression levels of genes related with the glutamate/aspartate pathway ( Supplementary Table 8 and Supplementary Note 2 ). With the exception of one AAT5 isoform missing in K326 but present in BX and TN90, we observed neither CNVs nor major transcriptomic variations, thereby suggesting that the nitrogen assimilation at the level of the glutamate/aspartate pathway is close between Burley tobacco and Flue-cured tobacco. However, it is not enough to conclude that the efficiency of ammonium assimilation is similar in both tobaccos, other downstream gene products from root to leaf being involved in the pathway as well as adaptations to environmental conditions. The analyses of the complete set of genes related to amino-acid assimilation will certainly help to understand the effect of human artificial selection on the high nitrogen requirement of Burley tobacco. Disease resistance TMV resistance was introduced in tobacco in the 1930s as a single dominant locus from an interspecific hybrid with Nicotiana glutinosa [42] , [43] , [44] . This locus was shown to harbour the N gene (NGU15605) encoding a (TIR)-NBS-LRR protein [45] that triggers a hypersensitive response following recognition of the viral helicase [46] . Among the three varieties sequenced here, only TN90 is TMV-resistant. TN90 has inherited the N gene from the variety Burley 21, which in turn inherited it from the variety Kentucky 56, which in turn inherited it from N. glutinosa hybrids [47] . Indeed, a search for the N. glutinosa N gene sequence in the draft assemblies showed weak identity in K326 and BX genomes (~90% identity on <35% of N. glutinosa genomic DNA), whereas a nearly perfect match was found for TN90 (99.9% identity over 7,158 bp). PVY is a potyvirus, which is transmitted by aphids, and has a broad host range including potato and tomato. N. tabacum is naturally susceptible to PVY and other potyviruses such as TVMV and TEV; interestingly, the ancestors N. tomentosiformis and N. sylvestris are resistant and susceptible, respectively, to PVY. Most modern tobacco varieties bred for PVY resistance carry alleles of the Va locus. The recessive va allele, which was first obtained by deletion [48] in the line TI 1406 (Virgin A Mutant) ( Supplementary Note 3 ), confers resistance by preventing virus cell-to-cell movement in a similar way to the recessive resistances of pepper, potato and tomato, suggesting the involvement of a eukaryotic initiation factor [49] . The characterization of the PVY resistance gene using a recombinant inbred line population was recently presented by Julio et al . [50] The eukaryotic translation initiation factor eIF4E was shown to be strongly expressed in susceptible plants, but not in resistant plants. We carried out a sequence comparison of the genome of TN90, which is resistant to the potyviruses TVMV, TEV and PVY, and the genomes of K326 and BX, which are susceptible. We identified eIF4E1 , eIF4E2 and eIF(iso)4E genes in the TN90, K326 and BX genome assemblies by first mapping corresponding tomato genes to N. sylvestris and N. tomentosiformis genomes, then mapping the respective genes to the tobacco genomes. One copy of each gene was found in the N. sylvestris genome, whereas two copies of eIF4E1 and one copy of the other genes were found in N. tomentosiformis . With the exception of the N. sylvestris eIF4E1 gene in TN90, all identified N. sylvestris and N. tomentosiformis genes were found in TN90, K326 and BX genomes. Gene-specific PCR verification ( Supplementary Fig. 7 ) showed that the absence of the N. sylvestris eIF4E1 in TN90 is not an artefact of genome assembly, but rather that it is missing from this variety. This confirms the observation that TVMV, TEV and PVY resistance in TN90 is caused by genomic deletion of the S-form eIF4E1 locus [50] . This is in line with the pattern of resistance observed in tobacco ancestors, suggesting that the dominant sensitivity of N. tabacum to potyviruses via the eIF4E1 mechanism was conferred by N. sylvestris . The fact that both S and T copies of N. tabacum eIF4E1 are expressed concomitantly ( Supplementary Table 9 ) allows us to speculate that either the interaction between the N. tomentosiformis eIF4E1 copies and viral proteins are compromised, or that the viral–host protein complex cannot provide the cell-to-cell movement required for systemic infection. Next-generation sequencing data were used to construct the genomes of three tobacco varieties, representing the three main market classes of commercially grown tobacco. Assembly accuracy was verified by mapping tobacco transcriptomics data, by assessing the consistency with tobacco physical and genetic maps, and through comparison of N. tabacum S- and T genomes to ancestral ( N. sylvestris and N. tomentosiformis ) genomes. The assemblies cover >80% of the genome, 75% being annotated as repeats. Sequencing and mapping of N. otophora in addition to mapping N. sylvestris and N. tomentosiformis genome sequences to the tobacco genomes confirmed that N. sylvestris and N. tomentosiformis are the most likely progenitors of N. tabacum . We observed a 4–8% genome reduction in the allotetraploid N. tabacum compared with its ancestral species. Between 81,000 and 94,000 gene models were identified for the three varieties. The alkaloid biosynthesis pathway characteristic of Nicotiana species and the glutamate/aspartate pathway did not show marked CNVs or preferential expression of genes from one ancestor within the investigated genes; indeed, only four of 32 identified homoeologous pairs were differentially expressed. This suggests that there was no adaptation affecting these two pathways at the genome or transcriptome level. The comparison of the genomes of the three varieties might shed some light on the effect of human selection, in addition to natural selection, resulting in resistance to TMV and potyviruses. However, more analyses about the evolution of R genes after the formation of allotetraploid will be necessary to understand this phenomenon. The draft genomes are sufficiently complete to both make and test hypotheses at the biological level, as exemplified by the analysis of virus resistance and alkaloid pathway genes. Together with the genome of N. otophora , they represent an important contribution to the SOL-100 genome project. Alongside genomes of the ancestral species N. sylvestris and N. tomentosiformis , the N. tabacum genome illustrates the evolutionary history of a complex allotetraploid. Finally, they strengthen N. tabacum as a plant model system, and as a platform for plant molecular farming. Plant material and nucleic acid isolation Seeds of N. tabacum TN90, K326 and Basma Xanthi ( Supplementary Note 4 ) were sterilized using chlorine gas and grown axenically on MS medium [51] for 4 months under artificial light (16 h day per 8 h night). DNA extraction was performed on aerial parts of one single plant of each variety using the Qiagen DNAeasy Plant Maxi Kit (Qiagen, Hilden, Germany). RNA extraction was performed using the Qiagen RNAeasy Mini Kit (Qiagen) on roots and leaves of three independent plants. In addition, nine TN90 tissues samples were analysed by the same method (see Supplementary Table 3 for details), whereby for 8 tissues biological triplicates were used and for one tissue biological duplicates were used. The DNA and RNA quantity and quality was verified using a Bioanalyzer (Agilent Technologies, Santa Clara, CA, USA). Genome and root and leaf transcriptome sequencing Short-insert ‘paired-end’ libraries were prepared using the Illumina TruSeq DNA Sample Preparation Kit version 2 (Illumina, San Diego, CA, USA). Long-insert ‘mate-pair’ libraries were prepared according to the Illumina Mate Pair Library Prep Kit version 2 (Illumina), or using a protocol developed by Fasteris SA (Geneva, Switzerland). In this case, 10 mg of genomic DNA was broken into fragments of ~2–5 kb using the Covaris E220 Focused-ultrasonicators (LGC Genomics, Berlin, Germany) and purified on a 0.7% agarose gel to recover 3 kb and 5 kb fragments. After ends-repair, a Fasteris-designed spacer was ligated and the fragments were circularized. After elimination of non-circular fragments, the DNA was again broken using the Covaris E220 Focused-ultrasonicators to generate fragments of 400 bp that were end-repaired ans ligated with Illumina adapters. RNA-seq libraries were constructed using the Illumina TruSeq RNA Sample prep Kit (Illumina). All libraries were sequenced on an Illumina HiSeq-2000 using version 3 chemistry and flow cells with runs of 2 × 100 bases. Base calling and sample demultiplexing were performed using Illumina HiSeq Control Software and CASAVA pipeline software. De novo genome assembly Raw DNA reads ( Supplementary Table 10 ) were preprocessed with FASTX toolkit utilities [52] by first trimming 3′ bases with qualities lower than 30, and then discarding reads shorter than 50 bases or with <90% of the bases with qualities lower than 30. The paired-end libraries with insert sizes shorter than 200 bases were further preprocessed using FLASH [53] to merge the paired-end reads into extended single reads. The paired and single reads from the paired-end libraries were then assembled into contigs using SOAPdenovo [27] with a k-mer of 63. Paired reads from paired-end and mate-pair libraries were used for scaffolding by increasing library size. To improve scaffolding, mate-pair libraries from the closely related Nicotiana species N. sylvestris and N. tomentosiformis [15] were also used ( Supplementary Table 11 ). SOAPdenovo was instructed to use these libraries only during its scaffolding step, and not during the building of contigs or during gap closing. Gaps resulting from the scaffolding were closed using GapCloser [27] and all sequences shorter than 200 bases were discarded from the final assemblies. After closing the gaps, singletons were blasted against the scaffolds and removed if matching was higher than 97% to avoid artificial duplication of short sequences. Figure 1 shows details of the N. tabacum TN90 genome. Synteny with other Solanaceae The tobacco assemblies were superscaffolded using the sequence-based WGP tobacco physical map. The obtained superscaffolds were then anchored to the tobacco genetic map by mapping of SSR markers. Synteny with the tomato and potato chromosomes ( Supplementary Data 2 and 3 ) was determined by mapping of tomato and potato reference proteins (ITAG2.3 and PGSC_DM_4.03) to the genetic map-anchored superscaffolds using BLAT [29] . The mapping was filtered to retain hits with at least 50% coverage and 80% identity. Supplementary Table 12 lists the number of proteins from each tomato and potato chromosome that are mapped to each linkage group. In addition to using the SSR markers shared between the N. tabacum , N. tomentosiformis and N. acuminata genetic maps, TAIR10 proteins for COSII markers present on two latter maps were also mapped with BLAT and filtered to retain hit with at least 50% coverage and 50% identity. To determine synteny between tomato or potato and tobacco using whole genomes ( Supplementary Data 4–7 ), we masked the genomes using tantan [54] , tandem repeat finder [55] and RepeatMasker and used nucmer [56] to detect syntenic DNA blocks. Analysis using MCScanX [32] was performed using the tomato and potato reference proteins and set of predicted proteins derived from the N. tabacum TN90 RNA-seq data ( Supplementary Data 8 and 9 ). Estimation of the quality of the assembly N. tabacum Hicks Broadleaf BAC sequences were sequenced by Roche 454 and assembled with newbler. In total 1,864,003 bases were obtained in sequences longer than 80 kb. The TN90, K326 and BX assemblies were mapped to these BACs sequences using blastn and a threshold of 98% identity, and the identified scaffolds remapped to the BAC sequences using LAST [57] , [58] . Repeat content estimation The repeat content of the genome assemblies was estimated using RepeatMasker with the eudicot repeat library available from the Sol Genomics Network, the TIGR Solanaceae repeat library and RepeatScout [59] libraries created using sequences of at least 200 kb from the draft genome assemblies. Classification of the repeat types was performed using blastn [60] hits to known repeat elements. Transcriptome assembly and quantitative analysis The transcriptomes were derived by mapping RNA-Seq reads from each variety to the corresponding reference genome. For each variety, three biological replicates were obtained for each tissue. Mapping was performed using the ‘tuxedo’ suite of short read mapping tools (Bowtie v2.0.0 beta [61] , Tophat v2.0.4 (ref. 62 ) and Cufflinks v2.0.2 (ref. 63 ). The resulting fragments were used as input for the Trinity software suite [64] open reading frame finder; the resulting predicted protein sequences were filtered for uniqueness and used for further analysis. GO terms were assigned to the unique subset of predicted protein sequences using InterProScan [38] . Protein clusters were determined using OrthoMCL [65] with standard parameters. Besides the predicted proteins from the TN90 transcriptome, we used the following sources to obtain proteins from other species: SGN for N. benthamiana , ITAG (version 2.3) for S. lycopersicum and TAIR (version 10) for A. thaliana . All protein sets were filtered for a minimum protein size of 100 amino-acid residues. For the quantitative analysis, the mapped RNA-seq reads were counted using HTSeq, and DESeq [66] was used to calculate differences in expression between the two tissues. Genes with a 10-fold upregulation and an associated adjusted P -value cutoff of 0.001 were deemed to be significantly differentially regulated. The set of overexpressed genes in leaves and roots was analysed for GO term enrichment. The software tool BiNGO [67] was used to calculate and visualize the enrichment. For determining enriched terms, the hypergeometric test was used with subsequent Benjamini and Hochberg false discovery rate corrections; a P -value threshold of 0.001 was used as a cutoff for inferring enrichment. Pathway gene identification Genes of interest were identified by mapping TAIR10 or UniProt proteins using BLAT [29] to the genomes of N. tabacum ancestors N. sylvestris and N. tomentosiformis [15] , extracting the identified genomic regions and 5 kb flanking regions, remapping the query protein using Exonerate [68] and predicting the target gene using SNAP [69] with the Exonerate hints. The thus-predicted N. sylvestris and N. tomentosiformis coding DNA sequences were then mapped to N. tabacum assemblies, and the N. tabacum coding DNA sequences and proteins were extracted using the above method. PCR eIF4 gene family detection Sequences related to eIF4E were identified by mapping tomato homologues as described above. In addition to the previously described PVY test primers [70] , specific primer pairs were designed for each eIF4E member ( Supplementary Table 13 ). Genomic DNA of different varieties was isolated as described in the plant section. PCR of genomic DNA was conducted using a 2-ng μl −1 template, 0.25 μM of each primer and GoTaq Hot Start polymerase (Promega AG, Switzerland). PCR was performed at 95 °C for 8 min, then 40 cycles of 30 s at 95 °C, 55 °C and 72 °C, sequentially, with a final extension at 5 min at 72 °C. PCR products were separated on a 1.2% agarose gel in 0.5 × TAE and visualized using ethidium bromide. Accession codes: Genome sequence data for Nicotiana tabacum TN90 has been deposited in DDBJ/EMBL/GenBank nucleotide core database under the accession code AYMY00000000. Genome and transcriptome sequencing data for N. tabacum TN90 have been deposited in GenBank Sequence Read Archive (SRA) under the accession code SRP029183 . Genome sequence data for Nicotiana tabacum K326 has been deposited in DDBJ/EMBL/GenBank nucleotide core database under the accession code AWOJ00000000. Genome and transcriptome sequencing data for N. tabacum K326 have been deposited in GenBank Sequence Read Archive (SRA) under the accession code SRP029184 . Genome sequence data for Nicotiana tabacum Basma Xanthi has been deposited in DDBJ/EMBL/GenBank nucleotide core database under the accession code AWOK01000000. Genome and transcriptome sequencing data for N. tabacum Basma Xanthi have been deposited in GenBank Sequence Read Archive (SRA) under the accession code SRP029185. Genome sequence data for Nicotiana otophora has been deposited in DDBJ/EMBL/GenBank nucleotide core database under the accession code AWOL00000000. Genome sequence data for N. otophora have been deposited in GenBank Sequence Read Archive (SRA) under the accession code SRP028836 . How to cite this article: Sierro, N. et al. The tobacco genome sequence and its comparison with those of tomato and potato. Nat. Commun. 5:3833 doi: 10.1038/ncomms4833 (2014).